Observation of an anomalous decoherence effect in a quantum bath at room temperature The decoherence of quantum objects is a critical issue in quantum science and technology. It is generally believed that stronger noise causes faster decoherence. Strikingly, recent theoretical work suggests that under certain conditions, the opposite is true for spins in quantum baths. Here we report an experimental observation of an anomalous decoherence effect for the electron spin-1 of a nitrogen-vacancy centre in high-purity diamond at room temperature. We demonstrate that, under dynamical decoupling, the double-transition can have longer coherence time than the single-transition even though the former couples to the nuclear spin bath as twice strongly as the latter does. The excellent agreement between the experimental and theoretical results confirms the controllability of the weakly coupled nuclear spins in the bath, which is useful in quantum information processing and quantum metrology. The coupling between a quantum object and its environment causes decoherence, which is a key issue in quantum science and technology [1] , [2] , [3] . Such coupling is usually understood in terms of classical noise, such as in the spectral diffusion theories that are widely used in, for example, magnetic resonance spectroscopy [4] , [5] and optical spectroscopy [6] , [7] . In modern nanotechnology and quantum science, the relevant environment of a quantum object can be of nanometre or even sub-nanometre size [8] , [9] , [10] , [11] , [12] , [13] , [14] , [15] , [16] , [17] , [18] , [19] , [20] , [21] , [22] . Therefore, the environment itself is quantum in nature. In recent years, quantum theories have been developed to treat the decoherence problem in a mesoscopic quantum bath [23] , [24] , [25] , [26] , [27] , [28] . These quantum theories have been successful in studying decoherence in various systems and predicted some surprising quantum effects [27] . A number of experiments have indicated the quantum nature of nuclear spin baths [8] , [10] , [11] , [12] , [16] , [17] . However, up to now, there has been no experiment explicitly addressing the fundamental difference between classical and quantum baths. A recent theoretical study [29] predicted an anomalous decoherence effect (ADE) of a quantum bath on a spin higher than 1/2. Considering a spin-1 under a unidirectional magnetic noise b z with Hamiltonian b z S z , the spin, initially in a superposition of the S z eigenstates | ψ (0)〉= a − |−〉+ a 0 |0〉+ a + |+〉, will evolve to | ψ ( t )〉= a − e iϕ ( t ) |−〉+ a 0 |0〉+ a + e iϕ ( t ) |+〉 with an accumulated random phase . The coherence of the single-transitions |0〉↔|±〉 is determined by the average of the random phase factor as L 0,± =〈 e ± iϕ ( t ) 〉, whereas the double-transition has coherence L −,+ =〈 e 2 iϕ ( t ) 〉. For Gaussian noise, as commonly encountered, L 0,± = e −〈 ϕ ( t ) ϕ ( t )〉/2 and L −,+ = e −2〈 ϕ ( t ) ϕ ( t )〉 = L 0,+ 4 . Decoherence of the double-transition behaves essentially the same as that of the single-transitions, but is faster as the double-transition suffers from noise that is twice as strong as that suffered by the single-transitions. Surprisingly, in a mesoscopic quantum bath made of nuclear spins, where the noise b z is the bath operator, the prediction is that the coherence time of the double-transition under dynamical decoupling, where the bath evolution is controlled through the flips of the central spin, can be increased above that of the single spin [29] . The nitrogen-vacancy (NV) centre in high-purity diamond, which has an electron spin-1 coupled to a nanometre-sized nuclear spin bath, is an ideal system to study the ADE. 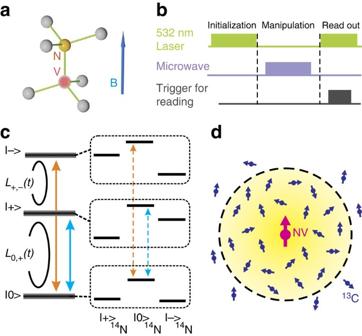Figure 1: System and methods for measuring NV centre spin decoherence in a13C nuclear spin bath in diamond. (a) Atomic structure of a nitrogen (N) - vacancy (V) centre in diamond and the magnetic fieldB. (b) Pulse sequences for the optically detected magnetic resonance measurement. The centre spin is initialized by the 532-nm laser pulse, manipulated by microwave pulses, and read out through the fluorescence. (c) Energy levels of an NV centre spin. The electron spin and14N-nuclear spin states are denoted by |ms〉 and |mI〉14Nforms,mI=0,±, respectively. The level splitting is caused by the hyperfine coupling to the14N nuclear spin. The single-transition coherenceL0,+and the double-transition coherenceL+,−are measured in the experiments. The solid (dashed) vertical arrows denote the nonselective (selective) microwave excitations of the centre spin. (d) Schematic of a13C-nuclear spin bath (enclosed by the circle), which together with the NV centre spin form a relatively closed quantum system. The NV centre electron spin (referred to as the centre spin hereafter; Figure 1a displays the structure) has long coherence time ( ∼ ms) even at room temperature [21] , and is promising for applications in quantum information processing [17] , [18] , [19] , [20] , [21] , [22] , [30] , [31] , [32] , [33] , [34] , [35] and nanometrology [36] , [37] , [38] , [39] , [40] , [41] . Besides the applications, the NV centre electron spin system is also a good model system for fundamental research on decoherence [28] , [29] and dynamical decoupling control [42] , [43] , [44] . The decoherence of NV centre electron spins in type-IIa samples is caused by coupling to the quantum spin bath formed from the 13 C nuclear spins that lie within several nanometres from the centre [28] , [29] . Figure 1: System and methods for measuring NV centre spin decoherence in a 13 C nuclear spin bath in diamond. ( a ) Atomic structure of a nitrogen (N) - vacancy (V) centre in diamond and the magnetic field B . ( b ) Pulse sequences for the optically detected magnetic resonance measurement. The centre spin is initialized by the 532-nm laser pulse, manipulated by microwave pulses, and read out through the fluorescence. ( c ) Energy levels of an NV centre spin. The electron spin and 14 N-nuclear spin states are denoted by | m s 〉 and | m I 〉 14N for m s ,m I =0,±, respectively. The level splitting is caused by the hyperfine coupling to the 14 N nuclear spin. The single-transition coherence L 0,+ and the double-transition coherence L +,− are measured in the experiments. The solid (dashed) vertical arrows denote the nonselective (selective) microwave excitations of the centre spin. ( d ) Schematic of a 13 C-nuclear spin bath (enclosed by the circle), which together with the NV centre spin form a relatively closed quantum system. Full size image Here we report the experimental observation of the ADE using an NV centre system at room temperature. The observed centre spin decoherence is in excellent agreement with the microscopic theory. The combined experimental and theoretical results demonstrate the capability of manipulating the evolution of the surrounding 13 C nuclear spins by controlling the centre spin. This manipulation paves the way for exploiting spin baths for quantum information processing [45] and nanometrology [39] , [41] . System and model We demonstrate the ADE using paramagnetic resonance measurements and microscopic calculations. The experiments are based on optically detected magnetic resonance [46] of single NV centres in type-IIa diamond at room temperature. After being polarized into the state |0〉 by a 532-nm laser pulse, the centre spin state is manipulated by the resonant microwave pulses and the spin coherence is read out through the measurement of fluorescence intensity ( Fig. 1b ). The calculation is based on a quantum many-body theory [26] , which takes into account the hyperfine coupling between the centre spin and the 13 C bath spins and the dipolar interaction between 13 C bath spins (see Methods). Under zero field, the centre spin has three eigenstates quantized along the z direction (the NV axis, [111] direction), namely, |±〉 and |0〉. In the experiment, a weak magnetic field (<20 gauss) is applied along the NV axis to lift the degeneracy between |+〉 and |−〉. Each energy level of the spin states |±〉 is split into three sub-levels owing to the hyperfine coupling with the 14 N nuclear spin in the NV centre ( Fig. 1c ). The coherence L 0,+ ( t ) of the single-transition |0〉↔|+〉 and the coherence L +,− ( t ) of the double-transition |+〉↔|−〉 ( Fig. 1c ) are measured for a single NV centre. The system has a Hamiltonian H = H NV + H B + H hf . The centre spin Hamiltonian is H NV =Δ S z 2 − γ e BS z , where Δ denotes the zero-field splitting and γ e =1.76×10 11 s −1 T −1 is the electron gyromagnetic ratio. The bath Hamiltonian contains the nuclear spin Zeeman splitting ( ω ) and the dipolar interaction between nuclear spins (with coefficients ). The centre spin couples to the nuclear spins through , where A j is the hyperfine coupling to the j th nuclear spin I j . Here the transverse components of the hyperfine coupling have been dropped because they are too weak to cause the centre spin flip (with A j <Δ). Owing to its dipolar form, the hyperfine coupling strength depends inverse-cubically on the distance of the nuclear spin from the centre. The relevant bath spins are those located within a few nanometres from the centre ( Fig. 1d ). Outside this range, the nuclear spins have too weak a hyperfine coupling to contribute to the centre spin decoherence [29] . Thus, within the decoherence timescale ( ∼100 bath spins form a relatively closed quantum system ( Supplementary Fig. S1 ). Free-induction decay of the centre spin coherence Viewed from the centre spin, the hyperfine coupling provides a quantum noise field . Since in general does not commute with the total Hamiltonian H , a certain noise-field eigenstate will evolve to a superposition of different eigenstates of , which leads to quantum fluctuations of the centre spin splitting. The Hamiltonian can also be expressed as where ω α =Δ− αγ e B is the eigenenergy of | α 〉, and governs the bath dynamics conditioned on the centre spin state. Viewed from the bath, the hyperfine coupling is a back action, conditioned on the centre spin state. Thus, the centre spin decoherence is caused by conditional bath evolution, which records the which-way information of the centre spin [25] , [29] . Besides the quantum fluctuations, there are also classical thermal fluctuations due to the random orientations of nuclear spins at room temperature. Indeed, the thermal fluctuations (also called inhomogeneous broadening) are much stronger than the quantum fluctuations and cause the free-induction decay of centre spin coherence within several microseconds. However, the inhomogeneous broadening effect can be removed by spin echo [47] . The coexistence of classical and quantum fluctuations and their different effects under spin echo control enable the in-situ comparison between the classical and quantum noises. 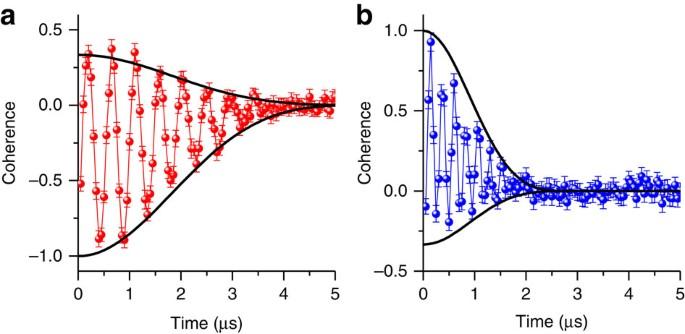Figure 2: Free-induction decay of the NV centre spin coherence. (a,b) Measured (colour lines with symbols) and calculated (envelopes in black lines) free-induction decay of the single- (a) and double-transition (b) coherence, respectively. The oscillations and the asymmetric envelopes are due to coupling to the14N nuclear spin. A magnetic fieldB=13.5 gauss is applied along the NV axis. Error bars are s.d. Figure 2 shows the free-induction decay of the centre spin coherence. Both single- and double-transition decoherence have Gaussian decay envelopes exp(− t 2 / T 2 *2 ), with the dephasing time of the double-transition ( T 2 * =1.16±0.11 μs) about half that of the single-transition ( T 2 * =2.33±0.39 μs). This verifies the scaling relation Figure 2: Free-induction decay of the NV centre spin coherence. ( a , b ) Measured (colour lines with symbols) and calculated (envelopes in black lines) free-induction decay of the single- ( a ) and double-transition ( b ) coherence, respectively. The oscillations and the asymmetric envelopes are due to coupling to the 14 N nuclear spin. A magnetic field B =13.5 gauss is applied along the NV axis. Error bars are s.d. Full size image as predicted in ref. 29 for thermal fluctuations. The experimental data are in good agreement with the numerical results obtained by considering the inhomogeneous broadening of a 13 C nuclear spin bath. Hahn echo of the centre spin coherence The quantum fluctuations become relevant when the inhomogeneous effect is removed by spin echo [47] . 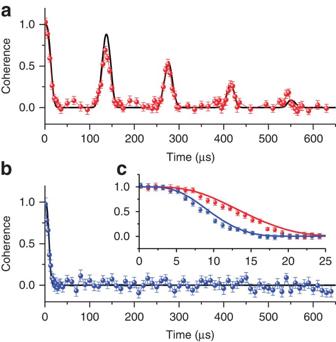Figure 3: Hahn echo of the NV centre spin coherence. (a,b) Measured (colour lines with symbols) and calculated (black lines) Hahn-echo signals of the single- (a) and the double-transition (b), respectively. (c) Close up of the initial decay in (a,b) for single- (red symbols for experiments and line for theory) and double-transition (blue symbols for experiments and line for theory). A magnetic fieldB=13.5 gauss is applied along the NV axis. Error bars are s.d. Figure 3 shows the Hahn echo signals under an external magnetic field B =13.5 gauss. The single-transition coherence presents periodic revivals. In contrast, the double-transition coherence decays to zero within several microseconds and does not recover. Such qualitative differences result directly from manipulation of the quantum bath on the centre spin flip. Figure 3: Hahn echo of the NV centre spin coherence. ( a , b ) Measured (colour lines with symbols) and calculated (black lines) Hahn-echo signals of the single- ( a ) and the double-transition ( b ), respectively. ( c ) Close up of the initial decay in ( a , b ) for single- (red symbols for experiments and line for theory) and double-transition (blue symbols for experiments and line for theory). A magnetic field B =13.5 gauss is applied along the NV axis. Error bars are s.d. Full size image Under a weak magnetic field, the centre spin decoherence is mainly induced by the single 13 C nuclear spin dynamics [28] , [39] , [48] . The dipolar interaction between nuclear spins can be neglected for the moment. Thus, the bath Hamiltonian H B only contains the nuclear Zeeman energy (with γ C B /2 π ∼ 14.4 kHz, γ C =6.73×10 7 s −1 T −1 being the gyromagnetic ratio of 13 C nuclei). The hyperfine field α A j (with A j /2 π ∼ 5 kHz for a nuclear spin I j located 1.5 nm from the centre) is comparable to the Zeeman frequency. Each nuclear spin precesses about different local fields h j ( α ) =− γ C B + α A j , conditioned on the centre spin state | α 〉. The centre spin decoherence is expressed as [28] , [39] , [48] . where | I j ( α ) ( t )〉 is the precession of the j th nuclear spin about the local field h j ( α ) starting from a randomly set initial state | I j 〉. The conditional evolution of bath spins records the which-way information of the centre spin and causes the decoherence. Under a flip operation of the centre spin | α 〉↔| α′ 〉, the nuclear spin precession is manipulated as , that is, the nuclear spin changes its precession direction and frequency. Thus, the nuclear spin bath is manipulated through control of the centre spin. The coherence at the echo time is calculated as [28] . When the centre spin is in the state |0〉, all the nuclear spins precess about the same local field B . This fact leads to the single-transition coherence recovery when the echo time is such that the nuclear spins complete full cycles of precession in a period of free evolution under the magnetic field (that is, γ C Bτ =2 nπ for integer n ). This effect is shown in Figure 3a , which is consistent with previous observations [17] . The height of the recovery peaks decays owing to the nuclear–nuclear spin interaction in the bath [28] , [39] , [48] ( Supplementary Fig. S2 ). For the double-transition coherence, however, the hyperfine couplings are non-zero and, therefore, the nuclear spins have different local fields for both of the centre spin states |±〉. Consequently, the double-transition coherence has no full recovery under the echo control in the weak field. Figure 3a,b show excellent agreement between the theory and the experimental observation. A close up of the initial coherence collapse (for γ C Bτ <2 π ) shows that the single-transition coherence still decays slower than the double-transition coherence ( Fig. 3c ). Actually, in the initial spin-echo decay under a weak magnetic field, the short time condition h j ( αα ) τ <1 is satisfied for most nuclear spins coupled to the centre spin. The short time expansion of equation (4) gives and which satisfy the scaling relation for classical Gaussian noise in equation (2) ( Supplementary Fig. S3 ). Thus, in the relatively short time range, the ADE is not yet fully developed. Dynamical decoupling control of the centre spin coherence To further explore the quantum nature of the nuclear spin bath, we employ the multi-pulse dynamical decoupling control, to elongate the centre spin coherence time and to make the control effects on the quantum bath more pronounced. 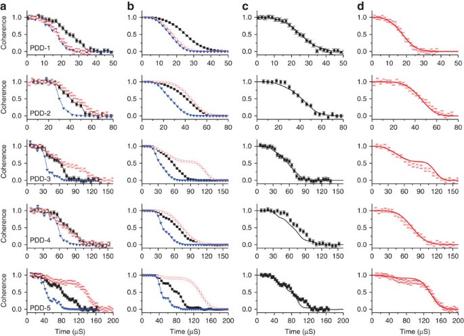Figure 4: Decoherence of the NV centre spin under PDD control. (a) Measured single- (black line with square symbols) and double-transition coherence (red line with circle symbols), under the one- to five-pulse PDD control (PDD-1 to PDD-5, from top to bottom). The scaled single-transition coherenceL0,+4(blue line with triangle symbols) is plotted for comparison. (b) The calculated data, plotted in the same format as in (a). (c) Comparison between the measured (symbols) and the calculated (solid lines) single-transition coherence. (d) The same asc, but for the double-transition. A magnetic fieldB=5 gauss is applied along the NV axis. Error bars are s.d. Figure 4 compares the single- and double-transition coherence under the periodic dynamical decoupling (PDD) control by equally spaced sequences of up to five pulses (applied at τ , 3 τ , 5 τ ..., called Carr–Purcell sequences for two or more pulses) [42] , [43] , [44] . To focus on the initial-stage decoherence, we use a weak field ( B =5 gauss) so that the subsequent revival of the centre spin coherence is suppressed since the revival period (about 0.37 ms in Hahn echo and 1.85 ms in PDD-5) is long as compared with the overall decoherence time [48] . In the Hahn echo (PDD-1), where the short time condition approximately holds, the single-transition coherence and the double-transition coherence approximately satisfy the scaling relation in equation (2). With increasing the number of control pulses, the double-transition coherence time increases more than that of the single-transition. Surprisingly, under the five-pulse control, the double-transition has significantly longer coherence time than the single-transition. Such counter-intuitive phenomena unambiguously demonstrate the quantum nature of the nuclear spin bath. Figure 4: Decoherence of the NV centre spin under PDD control. ( a ) Measured single- (black line with square symbols) and double-transition coherence (red line with circle symbols), under the one- to five-pulse PDD control (PDD-1 to PDD-5, from top to bottom). The scaled single-transition coherence L 0,+ 4 (blue line with triangle symbols) is plotted for comparison. ( b ) The calculated data, plotted in the same format as in ( a ). ( c ) Comparison between the measured (symbols) and the calculated (solid lines) single-transition coherence. ( d ) The same as c , but for the double-transition. A magnetic field B =5 gauss is applied along the NV axis. Error bars are s.d. Full size image The different dependence on dynamical decoupling of the single- and double-transition decoherence, though counter-intuitive, can be understood with a geometrical picture of nuclear spin precession conditioned on the centre spin state ( Fig. 5 ). By repeated flip control | α 〉↔| α′ 〉 of the centre spin, a nuclear spin I j precesses alternatively about the local fields h j ( α ) and h j ( α′ ) . The decoherence is caused mainly by the 13 C spins that are located close to the centre spin, which have hyperfine fields much stronger than the weak external field ( A j > γ C B ). The local fields h j (±) =− γ C B ± A j , corresponding to the centre spin states |±〉, are approximately anti-parallel and the bifurcated nuclear spin precession pathways have small distance δ +,− at echo time ( Fig. 5a displays a schematic of the evolution paths on the Bloch sphere, and Supplementary Movie 1 displays the animation). Thus, under dynamical decoupling control of the double-transition, the centre spin decoherence due to the closely located nuclear spins is largely suppressed. 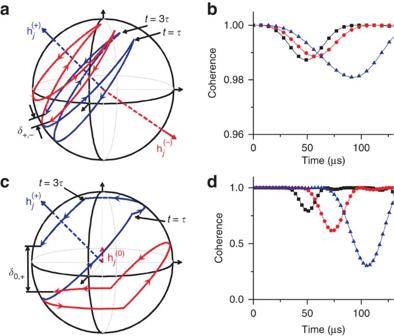Figure 5: Physical picture for understanding the ADE. (a) Bifurcated nuclear spin precession about the local fieldshj(+)(blue arrow) andhj(−)(red arrow) under the 2-pulse PDD control of the double-transition. The blue (red) path shows the nuclear spin precessing abouthj(+)(hj(−)) from time 0 toτfor the centre spin state |+〉 (|−〉), then precessing abouthj(−)(hj(+)) from timeτto 3τafter the centre spin is flipped to |−〉 (|+〉) at timeτ, and then precessing abouthj(+)(hj(−)) from time 3τto 4τafter the centre spin is flipped back to |+〉 (|−〉) at time 3τ. (b) The calculated decoherence of double-transition under PDD-5 control caused by three closely located13C spins in the randomly generated bath used in calculation forFigures 2,3,4. The coordinates (in units of lattice constant 0.357 nm) are (−3, −3, 5)/4, (2, 3/2, 1/2), and (1, −1, 2) for the black, red, and blue curves in turn. (c) The same as (a) but for the single-transition.δ+,−andδ0,+denote the distances between the bifurcated paths at the echo time (4τ) for the double- and single-transitions, respectively. As the two local fieldshj(±)are almost anti-parallel,δ+,−is much smaller thanδ0,+. (d) The decoherence of the single-transition due to the same three spins in (b). Notice the different scales of the vertical axes in (b,d). The contributions to the double-transition of these spins are much smaller than those to the single-transition. Figure 5b shows the contributions to the double-transition decoherence of three strongly coupled 13 C spins in the randomly generated spin bath (the same bath as used in calculation for Figures 2 , 3 , 4 ), which are largely suppressed by the dynamical decoupling control. On the contrary, this decoherence suppression mechanism does not exist in the single-transition case (Fig. 5c displays a schematic diagram of the evolution paths on the Bloch sphere and Supplementary Movie 2 displays the animation). Figure 5d shows the contributions to the single-transition decoherence of the same three strongly coupled 13 C spins as in Figure 5b , which are much greater than in the double-transition case. Thus, the overall coherence of the single-transition decays faster than that of the double-transition. This explains the ADE. Figure 5: Physical picture for understanding the ADE. ( a ) Bifurcated nuclear spin precession about the local fields h j (+) (blue arrow) and h j (−) (red arrow) under the 2-pulse PDD control of the double-transition. The blue (red) path shows the nuclear spin precessing about h j (+) ( h j (−) ) from time 0 to τ for the centre spin state |+〉 (|−〉), then precessing about h j (−) ( h j (+) ) from time τ to 3 τ after the centre spin is flipped to |−〉 (|+〉) at time τ , and then precessing about h j (+) ( h j (−) ) from time 3 τ to 4 τ after the centre spin is flipped back to |+〉 (|−〉) at time 3 τ . ( b ) The calculated decoherence of double-transition under PDD-5 control caused by three closely located 13 C spins in the randomly generated bath used in calculation for Figures 2 , 3 , 4 . The coordinates (in units of lattice constant 0.357 nm) are (−3, −3, 5)/4, (2, 3/2, 1/2), and (1, −1, 2) for the black, red, and blue curves in turn. ( c ) The same as ( a ) but for the single-transition. δ +,− and δ 0,+ denote the distances between the bifurcated paths at the echo time (4 τ ) for the double- and single-transitions, respectively. As the two local fields h j (±) are almost anti-parallel, δ +,− is much smaller than δ 0,+ . ( d ) The decoherence of the single-transition due to the same three spins in ( b ). Notice the different scales of the vertical axes in ( b , d ). The contributions to the double-transition of these spins are much smaller than those to the single-transition. Full size image Figure 4 shows excellent agreement between the measured centre spin decoherence under PDD and the calculation. Some features of slow oscillations or shoulders in the calculated decoherence do not perfectly match those in the measured data, especially for the higher order dynamical decoupling. This difference in the detail is understandable as such features are sensitive to the specific random positions of a few closely located 13 C spins, which are not determined. Nevertheless, the experiments unambiguously confirm the prediction that the double-transition coherence time grows to be longer than that of the single-transitions. Our observation of the ADE using NV centre coherence establishes the quantum nature of nuclear spin baths at room temperature. Previous studies of coherence control of NV centre spins in electron-spin baths [32] , [33] , [34] , [42] show that the decoherence is well described by classical noise theory. The fundamental difference between nuclear spin baths and electron spin baths lies in the intra-bath interaction strength relative to the bath-centre spin coupling [49] . For nuclear spin baths, the dipolar interaction between nuclear spins at average distance ( ∼ 10 Hz) is much weaker than the typical hyperfine coupling (>kHz) [28] , [29] . With such weak intra-bath interaction, the diffusion of coherence among nuclear spins is much slower than the decoherence (of a timescale ∼ ms). Thus, the centre spin and the bath can be regarded as a relatively closed quantum system. For electron spin baths, however, the coupling between bath spins at average distance is much stronger than the typical bath-centre coupling. As a result, the coherence will rapidly diffuse from closely located bath spins to those at distance during the centre spin decoherence. Therefore, an electron spin bath behaves like a macroscopic open system and the classical noise theory is valid. For NV centre spin decoherence in electron spin baths, we expect the ADE be absent and the scaling relation in equation (2) be observed instead. The quantum nature of nuclear spin baths can also be understood by the back-action of the centre spin to the bath. For the transition | α 〉↔| α′ 〉, the Hamiltonian in equation (1) can be expressed in a pseudo-spin form as , where σ z =| α 〉〈 α |−| α ′〉〈 α′ | is the pseudo-spin operator, b αα′ = H ( α ) − H ( α′ ) is the effective noise field to the pseudo-spin and is the effective bath Hamiltonian. For the single-transitions |0〉↔|±〉, the effective noise field is , and the double-transition |+〉↔|−〉 has a twice stronger noise as . For the double-transition, the effective bath Hamiltonian is H +− = H B , but for the single-transition the effective bath Hamiltonian is with the extra term owing to the hyperfine coupling, which is the back-action of the centre spin to the bath. For the nuclear spin bath, the hyperfine coupling is typically stronger than the intra-bath interactions and the back-action strongly modifies the effective bath Hamiltonian. In particular, for this work, the hyperfine coupling provides a much stronger local field than the applied magnetic field for nuclear spins close to the centre spin. In the single-transition case, because of the back-action, the nuclear spins have enhanced precession frequencies in comparison to the double-transition case. Thus, viewed from the centre spin, the effective bath for the double-transition produces noise with lower frequencies than in the single-transition case and, therefore, the centre spin coherence is better protected by the dynamical decoupling control. This explains the ADE observed in nuclear spin baths. In contrast, for electron spin baths, the coupling strength within the bath Hamiltonian H B is much larger than the back-action term (refs 32 , 33 , 34 , 42 , 49 ). For different centre spin transitions the modification of the bath dynamics due to the back-action is negligible. In this sense, the electron spin bath behaves as a classical bath and the ADE should not occur. Finally, we point out that, in this work, the ADE is demonstrated in the weak magnetic field regime (<20 gauss) in which the quantum fluctuations is caused mainly by single nuclear spin dynamics. The ADE was predicted in ref. 29 in the strong field regime, where the fluctuations are caused mainly by nuclear spin pair dynamics. These works indicate that the ADE is robust against the details of the decoherence mechanisms but is a universal phenomena due to the quantum nature of mesoscopic baths. Experimental setup All the experiments are carried out at room temperature. The type-IIa diamond single crystal sample has nitrogen density less than 5 ppb and the natural abundance of the 13 C isotope. Individual NV centres are optically addressed by a confocal microscope mounted on a piezoelectric scanner, and are identified by the measurement of the anti-bunching effect through the second-order correlation function ( Supplementary Fig. S4 ). To avoid the influence of the surface, an NV centre located 10 μm below the surface is used in the experiments. The weak magnetic field is generated by three pairs of Helmholtz coils with an accuracy of 1 degree for the direction and 0.01 gauss for the magnitude. All the pulse signals used in the experiments are synchronized by a pulse generator with time resolution of about 4 ns. Centre spin initialization and readout The centre spin state is initialized and read out by a 532 nm continuous-wave laser, which is gated using an acousto-optical modulator. A 10 μs optical pulse with an extra 5 μs waiting time pumps the system into the state |0〉. To read out the spin state, a 420 ns counting pulse is applied with a 620 ns waiting time after turning on the laser. Centre spin manipulation The centre spin is manipulated by resonant microwave pulses. A linear amplifier boosts microwave pulse power to the desired amplitude and a 20 μm diameter copper wire couples the microwave field into the diamond. The double-transition coherence is generated and controlled by composite pulses ( Fig. 6 ). The π /2-rotation of |+〉↔|−〉 is realized by a π /2-rotation of |0〉↔|+〉 followed by a π -rotation of |0〉↔|−〉, and the π -rotation of |+〉↔|−〉 is realized by two π -rotation of |0〉↔|−〉 sandwiched by a π -rotation of |0〉↔|+〉. For a fair comparison, the duration of a control in the single-transition coherence measurement is kept approximately the same as the total duration of the corresponding composite control in the double-transition coherence measurement. This is realized either by replacing π /2 and π rotations with 3 π /2 and 3 π rotations (amplitude kept the same but duration varied, Fig. 6a,b ), as in the experiments in Figures 2 and 3 where B =13.5 gauss, or by using pulses of smaller amplitudes in the single-transition coherence measurement ( Fig. 6c ), as in the experiments in Figure 4 where B =5 gauss. 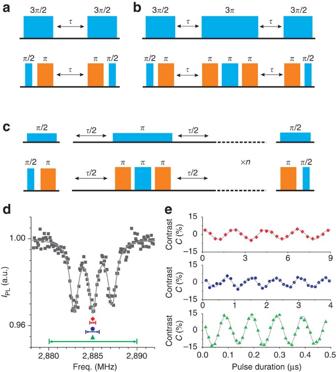Figure 6: Microwave manipulation of the centre spin. (a) Microwave pulse sequences for the free-induction decay experiments of single-transition (the upper sequence) and double-transition (the lower sequence) under 13.5 gauss magnetic field. The squares in blue (orange) represent the pulses that excite the |0〉↔|+〉 (|0〉↔|−〉) transition. The pulse areas are denoted above the squares. All the pulses are nonselective. (b) The same as (a), but for the Hahn echo measurements. (c) Microwave pulse sequences used in the PDD-nexperiments for the single-transition coherence measurement (the upper sequence) and those for the double-transition coherence measurement (the lower sequence) under 5 gauss magnetic field. The pulses are expressed in the same manner as in (a,b). Selective pulses are used to generate, control and read out the spin state. (d) The optically detected electron spin resonance spectrum of the |0〉↔|−〉 transition of the centre spin measured under 5 gauss magnetic field. The splitting due to the hyperfine coupling to the14N nuclear spin is resolved. The red, blue and green bars indicate, in turn, the three Rabi frequencies used in the experiments, 0.45 MHz (for selective excitation of single-transition inc), 1.3 MHz (for selective excitation of double-transition inc), and 10 MHz (for nonselective excitations ina,b). (e) From top to bottom, the Rabi oscillation with Rabi frequencies 0.45 MHz (selective excitation), 1.3 MHz (selective excitation), and 10 MHz (nonselective excitation), corresponding to the bars in (d). Figure 6: Microwave manipulation of the centre spin. ( a ) Microwave pulse sequences for the free-induction decay experiments of single-transition (the upper sequence) and double-transition (the lower sequence) under 13.5 gauss magnetic field. The squares in blue (orange) represent the pulses that excite the |0〉↔|+〉 (|0〉↔|−〉) transition. The pulse areas are denoted above the squares. All the pulses are nonselective. ( b ) The same as ( a ), but for the Hahn echo measurements. ( c ) Microwave pulse sequences used in the PDD- n experiments for the single-transition coherence measurement (the upper sequence) and those for the double-transition coherence measurement (the lower sequence) under 5 gauss magnetic field. The pulses are expressed in the same manner as in ( a , b ). Selective pulses are used to generate, control and read out the spin state. ( d ) The optically detected electron spin resonance spectrum of the |0〉↔|−〉 transition of the centre spin measured under 5 gauss magnetic field. The splitting due to the hyperfine coupling to the 14 N nuclear spin is resolved. The red, blue and green bars indicate, in turn, the three Rabi frequencies used in the experiments, 0.45 MHz (for selective excitation of single-transition in c ), 1.3 MHz (for selective excitation of double-transition in c ), and 10 MHz (for nonselective excitations in a , b ). ( e ) From top to bottom, the Rabi oscillation with Rabi frequencies 0.45 MHz (selective excitation), 1.3 MHz (selective excitation), and 10 MHz (nonselective excitation), corresponding to the bars in ( d ). Full size image With different pulse amplitudes under different magnetic field, the microwave pulse errors caused by coupling to the 14 N nuclear spin are greatly suppressed. Because of the hyperfine coupling to the 14 N nuclear spin, the microwave control is described by the Hamiltonian in the rotating-frame reference as H = A 0 S z I Z +√2 B 1 S x , where A 0 =2.18 MHz, is the hyperfine coupling strength and B 1 is the Rabi frequency of the driven field. Errors would result if the π pulses do not fully flip all the three hyperfine-split lines. Under a magnetic field B =13.5 gauss, a typical π pulse has a duration of 50 ns (corresponding to the Rabi frequency of about 10 MHz). Thus, the two centre spin single-transitions |0〉↔|±〉 are well resolved whereas the three transition lines for different states of the 14 N nuclear spin-1 are all spectrally covered ( Fig. 6d ). Under a magnetic field B =5 gauss it is difficult to spectrally resolve the two single-transitions without selection of different 14 N states. Therefore we use soft pulses (1.1 μs and 0.39 μs for the π-rotation in the single- and double-transition coherence measurements, respectively, corresponding to the Rabi frequencies of 0.45 MHz and 1.3 MHz) to selectively excite the single-transitions corresponding to only one of the 14 N states (namely the |0〉 14N state, Figure 6d ) and to maximally suppress the transitions when the 14 N nuclear spin is in the other two states (|±1〉 14N ). The selective and nonselective excitations are confirmed by the measurements of Rabi oscillations ( Fig. 6e ). The contrast measured by the selective pulse is one third of that measured by the nonselective pulse. Data processing and error analysis The measured contrast is given by the relative change in fluorescence intensity as C =( I M − I ∞ )/ I 0 , where I M is the signal, I ∞ is the fluorescence where the spin coherence has totally decayed and I 0 is the fluorescence when the centre spin is in the state |0〉, all of which are measured independently in every experimental run. The contrast is normalized to the averaged value at the initial decoherence stage (for small time, where the coherence presents the plateau feature). The results, however, do not depend on the normalization ( Supplementary Fig. S5 ). The statistical errors come mainly from the photon-counting shot noises and laser-focusing spot drifting. To suppress errors from the laser-focus drifting, the laser is re-focused every 20 min during the measurement. To reduce the effect of the shot noises, each measurement has been repeated about 10 6 times. The background photon counting I 0 is measured by more than 10 7 times so that its statistical fluctuation can be neglected. Besides the statistical fluctuations, there are two major causes of systematic errors: first, the MW pulse frequencies are determined with an error about ±20 kHz, less than 4% of the Rabi frequencies; and second, the durations of the pulses are determined up to an error of ±2 ns, which induces an error in the Rabi frequencies of about 4% in the case of short control pulse used in the experiments in Figures 2 and 3 (where the π pulses have durations of about 50 ns), but has negligible effect in the case of soft control pulse used in the experiments in Figure 4 . The above factors contribute to the error bars estimated and shown in Figures 2 , 3 , 4 . Theoretical model and numerical simulation methods In the numerical calculation, the nuclear spin bath is generated by randomly placing 13 C atoms on the diamond lattice around the NV centre with a natural abundance 1.1%. Inclusion of about 100 13 C nuclear spins within 2 nm from the NV centre is sufficient for a converged result of the centre spin decoherence in the timescale considered in this paper. The inhomogeneous broadening and decoherence times depend on the random positions of the 13 C atoms in the lattice [28] , [48] . In the simulation, the configuration of 13 C atom positions is randomly chosen to produce a single-transition dephasing time T 2 * and a single-transition decoherence time in Hahn echo ( T 2 ) close to the experimental results (under 13.5 gauss field). Otherwise, there is no fitting parameter. Different random configurations of the 13 C atom positions do not affect the essential results but result in differences in the detailed features ( Supplementary Fig. S6 ). The generated bath does not contain a 13 C in the first few coordinate shells of the NV centre (which has hyperfine coupling >1 MHz), to be consistent with the NV centre under the experimental observation. The hyperfine interaction is assumed to have a dipolar form with the electron spin located at the vacancy site. The spin coherence is calculated by applying the cluster correlation expansion method [26] , which takes into account, order by order, the many-body correlations induced by the dipolar interactions between nuclear spins, and can identify the contribution of each nuclear spin cluster to the total decoherence. The converged results are obtained by including clusters containing up to 3 nuclear spins. The microwave pulses are modelled by instantaneous pulses, which is a good approximation considering the fact that the pulse durations are all much shorter than the decoherence times in the experiments. How to cite this article: Huang, P. et al . Observation of an anomalous decoherence effect in a quantum bath at room temperature. Nat. Commun. 2:570 doi: 10.1038/ncomms1579 (2011).